A stem-group cnidarian described from the mid-Cambrian of China and its significance for cnidarian evolution Palaeontological data of extinct groups often sheds light on the evolutionary sequences leading to extant groups, but has failed to resolve the basal metazoan phylogeny including the origin of the Cnidaria. Here we report the occurrence of a stem-group cnidarian, Cambroctoconus orientalis gen. et sp. nov., from the mid-Cambrian of China, which is a colonial organism with calcareous octagonal conical cup-shaped skeletons. It bears cnidarian features including longitudinal septa arranged in octoradial symmetry and colonial occurrence, but lacks a jelly-like mesenchyme. Such morphological characteristics suggest that the colonial occurrence with polyps of octoradial symmetry is the plesiomorphic condition of the Cnidaria and appeared earlier than the jelly-like mesenchyme during the course of evolution. The basal metazoan phylogeny is one of the most intractable problems in animal evolution. Diverse views have been presented to address the relationships among the basal metazoan groups including the Porifera, Cnidaria, Placozoa, Ctenophora and Bilateria [1] , [2] , and to date no consensus on the origin of each of these groups has been reached. Palaeontological data have frequently contributed to revealing the metazoan evolution [3] , [4] , [5] , [6] , [7] , [8] , [9] , [10] , but fossils which would have provided crucial information on the origin of the Cnidaria have not hitherto been documented. A few Ediacaran fossils have been referred to cnidarians [11] , [12] , but have not been proven to be stem-group cnidarians. In fact, the cnidarian affinity of many Ediacaran fossils has been questioned [13] , [14] . The Cambrian fossils of unequivocal cnidarian affinity are placed within the crown-group cnidarians [15] , [16] , [17] , [18] , [19] , hence failing to provide any useful insight on the origin of the Cnidaria. In this study, we report exquisitely preserved fossils of a stem-group cnidarian, C. orientalis gen. et sp. nov., from the mid-Cambrian Changhia Formation in Shandong Province, China, and discuss its implication for the evolutionary origin of the Cnidaria. Systematic palaeontology Stem-group Cnidaria Cambroctoconus gen. nov. Etymology . The generic name refers to the Cambrian octagonal conical cup-shaped organism. Type species . C. orientalis sp. nov. Diagnosis . Colony composed of calcareous conical cup-shaped skeletons. Individual cup eight-sided, with holdfast; cup opening octagonal in plan view. Pair of longitudinal lamellar septa project inwards from each corner of the cup. Wall perforated. Cambroctoconus orientalis sp. nov. Etymology . From Orientalis , Latin for eastern, referring to the occurrence in eastern Asia. Holotype . Seoul National University palaeontological collection no. SNUP7001 ( Fig. 1a ). Locality and horizon . Three localities in Shandong Province, China ( Supplementary Fig. S1 ); middle part of the Changhia Formation. Specimens of the Mantoushan section are calcareous, whereas those of the Jiulongshan and Xintai sections are partly silicified. All of the specimens are collected from the stratigraphically equivalent horizons. Age . Crepicephalina zone; Drumian stage (Cambrian Series 3). Diagnosis . As for the generic diagnosis. 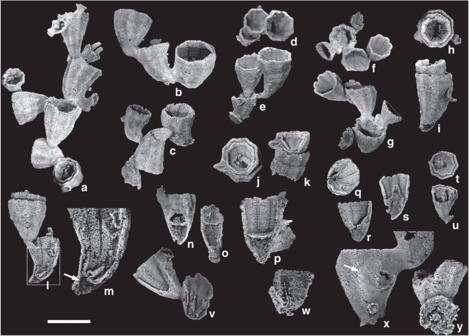Figure 1:Cambroctoconus orientalisfrom the mid-Cambrian Changhia Formation in Shandong Province. All specimens are silicified and etched out by hydrochloric acid. (a) SNUP7001, holotype, comprising more than 10 individuals. Note the small circular structures on the surface of the cups, which represent incipient offsets. (b) SNUP7002, with three individuals. (c) SNUP7003, note that the growing direction of the offsets is opposite to that of the parental cup. (d,e) SNUP7004, two offsets grew from an incompletely grown parental cup. (d) Plan view. (e) Lateral view. (f,g) SNUP7005, two offsets budded from the rim of the parental cup. (f)Plan view. (g) Lateral view. (h,i) SNUP7007, an offset grown from the inside of the parental cup. (h) Plan view. (i) Lateral view. (j,k) SNUP7008, a specimen displaying a longitudinal cut view of a small offset. (j) Plan view. (k) Lateral view. (l,m) SNUP7009, a specimen displaying a longitudinal cut view of the parental cup with a tubular structure at its base. The dotted rectangle is magnified in (m) to show the basal cavity and tubular structure (white arrow). (n,o) SNUP7010, partly broken cup showing the subhorizontal element and basal cavity. Two pieces are complementary to each other. (p) SNUP7011, specimen with subhorizontal element. (q,r) SNUP7013, a partially broken specimen showing clearly impressed growth lines. Vertical depressions represent the position of paired septa at corners. (q) Plan view. (r) Partly cut lateral view. (s–u) Specimens with a conical protuberance. (s) SNUP7014, longitudinal-cut view. (t,u) SNUP7015. (t) Plan view. (u) Partly cut lateral view. (v) SNUP7016, specimen with two tubular structures, longitudinal-cut view. (w) SNUP7017, a fragmentary specimen showing incompletely preserved septa. (x) SNUP7018, a specimen with a holdfast of the offset on the parental cup (white arrow). Note that the holdfast of the offset is solid and clearly distinguished from the perforated wall of the parental cup. (y) SNUP7019, a detached cup showing the base of the holdfast. The scale bar is 10 mm fora–v(exceptm), and 5 mm forw–y. Figure 1: Cambroctoconus orientalis from the mid-Cambrian Changhia Formation in Shandong Province. All specimens are silicified and etched out by hydrochloric acid. ( a ) SNUP7001, holotype, comprising more than 10 individuals. Note the small circular structures on the surface of the cups, which represent incipient offsets. ( b ) SNUP7002, with three individuals. ( c ) SNUP7003, note that the growing direction of the offsets is opposite to that of the parental cup. ( d , e ) SNUP7004, two offsets grew from an incompletely grown parental cup. ( d ) Plan view. ( e ) Lateral view. ( f , g ) SNUP7005, two offsets budded from the rim of the parental cup. ( f) Plan view. ( g ) Lateral view. ( h , i ) SNUP7007, an offset grown from the inside of the parental cup. ( h ) Plan view. ( i ) Lateral view. ( j , k ) SNUP7008, a specimen displaying a longitudinal cut view of a small offset. ( j ) Plan view. ( k ) Lateral view. ( l , m ) SNUP7009, a specimen displaying a longitudinal cut view of the parental cup with a tubular structure at its base. The dotted rectangle is magnified in ( m ) to show the basal cavity and tubular structure (white arrow). ( n , o ) SNUP7010, partly broken cup showing the subhorizontal element and basal cavity. Two pieces are complementary to each other. ( p ) SNUP7011, specimen with subhorizontal element. ( q , r ) SNUP7013, a partially broken specimen showing clearly impressed growth lines. Vertical depressions represent the position of paired septa at corners. ( q ) Plan view. ( r ) Partly cut lateral view. ( s – u ) Specimens with a conical protuberance. ( s ) SNUP7014, longitudinal-cut view. ( t , u ) SNUP7015. ( t ) Plan view. ( u ) Partly cut lateral view. ( v ) SNUP7016, specimen with two tubular structures, longitudinal-cut view. ( w ) SNUP7017, a fragmentary specimen showing incompletely preserved septa. ( x ) SNUP7018, a specimen with a holdfast of the offset on the parental cup (white arrow). Note that the holdfast of the offset is solid and clearly distinguished from the perforated wall of the parental cup. ( y ) SNUP7019, a detached cup showing the base of the holdfast. The scale bar is 10 mm for a – v (except m ), and 5 mm for w – y . Full size image Description Individual cups are usually 11–13 mm in height, 8–11 mm in maximum width near the rim and 1.5–3 mm in minimum width near the base ( Figs 1 , 2 , 3 ). The base expands to form a holdfast. The lower part of the cup is generally curved in the offsets budded from the outer surface of the parental cup ( Fig. 1b–e ), but straight in those budded from the rim ( Fig. 1f,g ). The wall is perforated, except for the holdfast ( Figs 1x and 2 ). Paired longitudinal septa project inwards from each corner ( Figs 1w and 2b–d ; Supplementary Fig. S2 ). The septa appears to be perforated ( Fig. 2b–d ). Transverse growth lines are expressed on the inner surface of the cup ( Fig. 1p–r ). A hollow space in the lowermost part of the cup may represent a basal cavity ( Figs 1l–p,w , 2f,h , 3a,c–p ; Supplementary Fig. S3h ). The top of the basal cavity is occasionally defined by a subhorizontal element ( Fig. 1n–p ), which is located as high as one-half of cup height. Longitudinal septa extend downwards to the subhorizontal element ( Fig. 1l–p ), implying that the gastrovascular cavity, if present, would have been placed on this structure. The internal base of the cup also displays some peculiar structures such as conical protuberance ( Figs 1s–u , 2f , 3d–p ) and tubular structures ( Fig. 1l,m,v ). 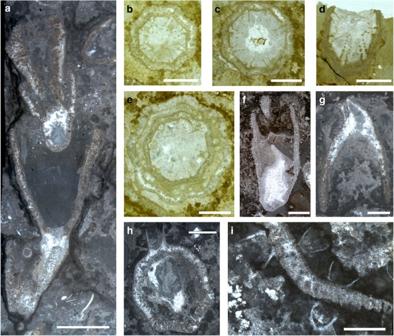Figure 2: Thin-section photographs ofCambroctoconus orientalis. (a) SNUP7020, longitudinal section of four individuals. The second offset from the bottom budded from the rim of the parental cup. The topmost offset budded from the internal base of the parental cup. Scale bar is 5 mm. (b–e) Transverse views of cups, showing the eight-paired septa. (b) SNUP7021. Scale bar is 2 mm. (c) SNUP7022. Scale bar is 2 mm. (d) SNUP7023, note that some septa are apparently perforated. Scale bar is 2 mm. (e) SNUP7024, parental cup (outer one) and its offset (inner one). Scale bar is 2 mm. (f) SNUP7025, longitudinal section of a cup, which displays the conical protuberance and basal cavity at the base. Scale bar is 5 mm. (g) SNUP7026, a pendant individual with subhorizontal element. Scale bar is 2 mm. (h) SNUP7027, an offset budded from the outer surface of the parental cup. Scale bar is 2 mm. (i) SNUP7028, offsets budded from both inner and outer surfaces of the parental cup. Scale bar is 1 mm. Figure 2: Thin-section photographs of Cambroctoconus orientalis . ( a ) SNUP7020, longitudinal section of four individuals. The second offset from the bottom budded from the rim of the parental cup. The topmost offset budded from the internal base of the parental cup. Scale bar is 5 mm. ( b – e ) Transverse views of cups, showing the eight-paired septa. ( b ) SNUP7021. Scale bar is 2 mm. ( c ) SNUP7022. Scale bar is 2 mm. ( d ) SNUP7023, note that some septa are apparently perforated. Scale bar is 2 mm. ( e ) SNUP7024, parental cup (outer one) and its offset (inner one). Scale bar is 2 mm. ( f ) SNUP7025, longitudinal section of a cup, which displays the conical protuberance and basal cavity at the base. Scale bar is 5 mm. ( g ) SNUP7026, a pendant individual with subhorizontal element. Scale bar is 2 mm. ( h ) SNUP7027, an offset budded from the outer surface of the parental cup. Scale bar is 2 mm. ( i ) SNUP7028, offsets budded from both inner and outer surfaces of the parental cup. Scale bar is 1 mm. 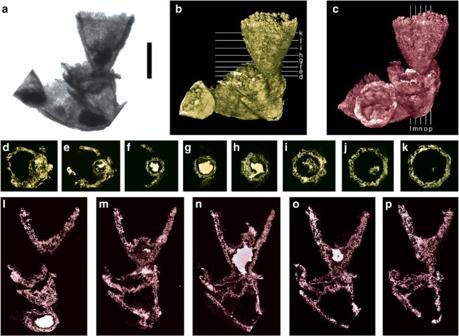Figure 3: Micro-CT images ofCambroctoconus orientalisSNUP7051. (a) A projection image of SkyScan1172. The portion with higher density of the skeleton is represented darker in the image. The internal cavity of the skeleton is filled with precipitated silica, hence higher in density. Scale bar is 5 mm. (b,c) 3-D reconstructions with white lines indicating the horizontal and perpendicular surfaces, which are shown ind–kandl–p, respectively. The cavity-filling silica is represented with a bright colour ind–p. Note that the individual represented ind–ppossesses a conical protuberance. Full size image Figure 3: Micro-CT images of Cambroctoconus orientalis SNUP7051. ( a ) A projection image of SkyScan1172. The portion with higher density of the skeleton is represented darker in the image. The internal cavity of the skeleton is filled with precipitated silica, hence higher in density. Scale bar is 5 mm. ( b , c ) 3-D reconstructions with white lines indicating the horizontal and perpendicular surfaces, which are shown in d – k and l – p , respectively. The cavity-filling silica is represented with a bright colour in d – p . Note that the individual represented in d – p possesses a conical protuberance. Full size image All new offsets bud from the parental cups by asexual reproduction. The offsets start as small circular structures that occur randomly at the cup surface ( Fig. 1a,b,e,i,x ), and then grow upwards and outwards. Most offsets bud from the outer surface of the cup ( Figs 1a–e , 2h,i ; Supplementary Fig. S3b,e,h,i,l ), but some bud from the inner surface ( Figs 1h–l , 2a,e,i ) and others even from the rim ( Figs 1f,g , 2a ). Those offsets budded from the inner surface of the parental cup exhibit a strong coordination in keeping the octagonal shape, showing a double-walled appearance ( Figs 1h,j , 2e ; Supplementary Fig. S3d ). Individuals budded from the rim of the parental cup have a holdfast that incompletely wraps around the rim ( Fig. 1g ). Most offsets are oriented in the same direction as the parental cup ( Fig. 1b,d,e ), while some are oriented in the opposite direction ( Fig. 1c ). In general, adjacent cups are aligned in a certain direction to form crudely lobed clusters in a colony ( Supplementary Fig. S4 ). Life mode Although orientation of the cup is rather random, the colony appears to have grown laterally as a whole ( Supplementary Figs S4, S5 ). The colonial development is not as strictly regular as in the extant Anthozoa, but the lobes are oriented roughly into two directions, displaying a sort of branching pattern within the colony. The colony is further differentiated from that of the Anthozoa, in that it lacks the shared colonial tissue (coenenchyme). Eight pairs of longitudinal septa are reminiscent of those of the crown-group cnidarians. However, in case of the offset budded from the inner surface, the internal space of the parental cup cannot have functioned properly, as most of the space was taken by the offset. Therefore, whichever function related to the internal space of the parental cup, must have been restricted to accommodate the offset. The association of microbes and small sponges in the bioherms indicates that C . orientalis lived in a shallow water environment. In a collection from the Xintai section, some individuals face their cup opening downwards, as if they were pendent from the flank of the microbial bioherm in life ( Fig. 2g ; Supplementary Fig. S3g,i,j ). They might have dwelled in shaded or possibly in cryptic habitats. A range of orientation of the offsets ( Fig. 1a,c ; Supplementary Fig. S3 ) suggests that their growth directions, in general, would not have been strongly influenced by external factors such as light or currents. C. orientalis possesses cnidarian features such as the longitudinal septa and octoradial symmetry, as well as non-cnidarian features such as the perforated wall and basal cavity. A cladistic analysis places Cambroctoconus as a stem-group cnidarian ( Fig. 4 ). The phylogenetic position of C . orientalis as a stem-group cnidarian coupled with the morphological comparison of C . orientalis with such extant cnidarians as octocorals and staurozoans, sheds light on the evolutionary sequences of the Cnidaria. The Octocorallia is the most basal group of the Anthozoa [20] , [21] , [22] , which has been recently interpreted as the most basal group of the Cnidaria [20] , [23] , [24] . The octocorals are colonial and have eight mesenteries within the gastrovascular cavity and eight tentacles around the mouth. It is noteworthy that the eight mesenteries and eight tentacles of the octocorals are arranged in an octoradial symmetry as are the eight-paired septa and eight-sided cup of C . orientalis , and both organisms are colonial. The Staurozoa is placed between the Anthozoa and the Medusozoa in recent phylogenetic analyses using molecular data [20] , [25] . The staurozoan is conical cup-shaped and solitary in occurrence, and has eight tentacle-bearing arms around the mouth and a holdfast-like attachment disc at the base, displaying resemblance to an individual cup of C. orientalis . 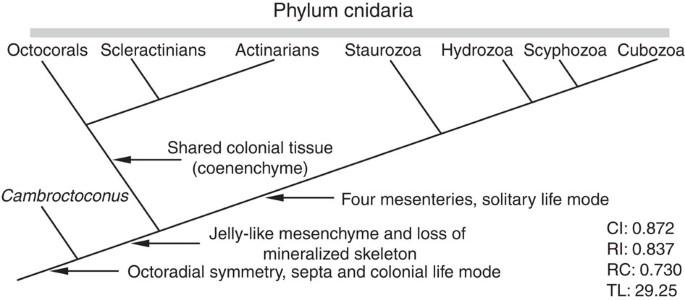Figure 4: Outline of cnidarian phylogeny displaying stem-group position ofCambroctoconus orientalis. The topology is 1 of the 24 trees generated by the initial analysis, which is also found out of the 12 trees obtained by the character-reweighted second run. The tree scores are from the second run. The topology within the crown group cnidarians is consistent with the recent cnidarian tree, based on the molecular data20. CI, consistency index; RI, retention index; RC, rescaled consistency index; TL, tree length. Figure 4: Outline of cnidarian phylogeny displaying stem-group position of Cambroctoconus orientalis . The topology is 1 of the 24 trees generated by the initial analysis, which is also found out of the 12 trees obtained by the character-reweighted second run. The tree scores are from the second run. The topology within the crown group cnidarians is consistent with the recent cnidarian tree, based on the molecular data [20] . CI, consistency index; RI, retention index; RC, rescaled consistency index; TL, tree length. Full size image Budding of new individuals in the crown-group cnidarians invariably occurs in the soft part of polyps. In particular, the anthozoan polyps are embedded in and arise from a mass of jelly-like mesenchyme (mesoglea+some cell products) [26] , which occurs between epidermis and gastrodermis. In contrast, the offsets of C. orientalis budded from both inner and outer surfaces of the skeletal cup, implying that C. orientalis must have possessed a skeletal wall highly integrated with soft tissue of the animal from which new offsets could arise. This is in contrast to the exoskeletons of other extinct and extant cnidarians, which are generally epitheca, not highly integrated with soft tissue of the polyps. Therefore, even if C. orientalis possessed a mesenchyme-equivalent structure, it cannot have been jelly-like structure as present in the known cnidarians. As the jelly-like mesenchyme is present in all crown-group cnidarians, its absence in C. orientalis indicates that octoradial symmetry, septa and colonial life mode appeared earlier than jelly-like mesenchyme in the course of cnidarian evolution ( Fig. 4 ). The morphological comparison leads us to reconstruct the plesiomorphic cnidarians as follows: the polyp is a conical cup with attachment disc, but probably without mineralized skeleton; each polyp has eight tentacles and eight mesenteries; and the polyps form a colony that lacks coenenchyme. This primitive form evolved into two cnidarian branches: one leading to the anthozoans that developed coenenchyme and the other to staurozoans/medusozoans that reduced the number of mesenteries to four and lost the colonial mode of life ( Fig. 4 ). Fossil localities Fossils of C. orientalis were collected from the mid-Cambrian Changhia Formation at three localities in Shandong Province: the Mantoushan section (36° 25′ 45′′ N, 116° 53′ 53′′ E), the Jiulongshan section (36° 04′ 51′′ N, 117° 44′ 18′′ E) and the Xintai section (35° 45′ 05′′ N, 117° 46′ 22′′ E) ( Supplementary Fig. S1 ). The Changhia Formation is a thick succession of oolitic and microbial carbonates, which were deposited in a shallow carbonate platform. This stem-group cnidarian occurs in the thrombolitic and dendrolitic microbial bioherms in association with calcified microbes (for example, Epiphyton ) and anthaspidellid sponges. Preparation of specimens Serial thin sections were made for the samples from all three localities. Silicified specimens from the Jiulongshan and Xintai sections were dissolved out by hydrochloric acid and/or acetic acid. As the specimens from the Mantoushan section have exclusively calcareous skeleton, only thin sections were made, without any chemical treatment. The chemical treatment of the Xintai material produced a better result than the Jiulongshan material. Many specimens were detached from the colony during the chemical treatment. The detached specimens were coated with magnesium oxide and are illustrated in Figure 1 . The specimens left in the partially dissolved-out colony are illustrated in Supplementary Figure S6 . The X-ray microcomputed tomography scan was carried out using the SkySkan 1172 system at the Dental Research Institute of Seoul National University. The skeleton was scanned with beam energy of 80 keV and a flux of 124 μA at a detector resolution of 12.97 μm per pixel using a 180° rotation with a step size of 0.4°. To reconstruct the images of Figure 3b–p , 481 transmission images were reconstructed in a 2,000×2,000 matrix of 1,046 slices. Figure 3b and c were reconstructed with a resolution of 12.97 μm per voxel using the SkyScan software CTVox32. Figures 3d–p were acquired with the SkyScan software DataViewer. Chemical composition of skeleton The chemical composition of the skeleton of C. orientalis from three different localities was analysed by Energy Dispersal Spectrometry. Specimens from the Mantoushan section retain the original calcareous skeleton ( Supplementary Table S1 ), whereas those from the Jiulongshan section have been partially silicified ( Supplementary Table S2 ) and those from the Xintai section have been heavily silicified ( Supplementary Table S3 ). Cladistic analysis Overall, 28 characters were coded for ten taxa including two multiple outgroups (see Supplementary Table S4 for character matrix and character and state description). Among these, 16 characters were obtained from a pre-existing character matrix of a phylogenetic analysis of the Cnidaria [27] . In the original character matrix [27] , 87 characters were coded for 15 taxa (Anthozoa, Staurozoa, Conulatae, Cubozoa, three scyphozoan orders and eight hydrozoan orders). As the Scyphozoa and the Hydrozoa were herein treated as a single taxon, respectively, those characters that are only informative for the relationship within each group were not included. Uninformative characters were also excluded. All characters were equally weighted and unordered in the initial run. There is no consensus on the relationship among the basal metazoans including the Porifera, Cnidaria, Placozoa, Ctenophora and Bilateria [1] , [2] . Recent analyses using molecular data provide inconsistent results: some generate a clade of the Porifera and Cnidaria [28] , [29] , [30] , [31] , whereas others generate a nested pattern in which the Placozoa and/or Ctenophora are placed between the former two groups [23] , [24] , [32] . Given the uncertainty of the basal metazoan phylogeny, the Porifera and Placozoa were selected as multiple outgroups, but it does not necessarily mean that the two groups are phylogenetically closer to Cnidaria than to Ctenophora and Bilateria. Although the conical cup-shaped skeleton of C. orientalis resembles the skeleton of archaeocyathans, an extinct poriferan group, in having a perforated conical cup-shaped skeleton, the octoradial symmetry and paired longitudinal septa are not archaeocyathan features. Moreover, archaeocyathans suffered a major extinction at the end of the lower Cambrian, and are hardly known from the middle Cambrian strata [33] . We, therefore, do not consider that C. orientalis is closely allied to archaeocyathans. The phylogenetic analysis was performed using PAUP 4.0 b 10 (ref. 34 ). The exhaustive search option was used to produce the most parsimonious trees. Unavailable and inapplicable character states are coded as '?' and '-', respectively. Polymorphic characters are coded as '0/1'. The matrix was calculated using the exhaustive search under ACCTRAN option with random stepwise-addition condition of 1000 replicates and 100 trees held at each step. A total of 24 maximum parsimonious trees was obtained by the initial run with the tree-length of 35: consistency index is 0.800; retention index is 0.741; and rescaled consistency index is 0.593. The strict consensus tree of the 24 most parsimonious trees results in a polytomy of all in-group taxa. Then, the characters were weighted by their rescaled consistency index, and were analysed with the heuristic search, which generated 12 most parsimonious trees with the tree length of 29.25: consistency index is 0.872; retention index is 0.837; and rescaled consistency index is 0.730. The strict consensus tree and 50% majority rule tree of the 12 trees are shown in Supplementary Figures S7 and S8 , respectively. Nine of the twelve trees place Cambroctoconus under the crown group cnidarians as a stem-group ( Supplementary Fig. S8 ); other three trees position Cambroctoconus as the basal branch of the Anthozoa. Figure 4 shows a topology of a tree that is generated from both analyses and is consistent with the recent molecular phylogeny [20] . How to cite this article: Park, T.-y. et al . A stem-group cnidarian described from the mid-Cambrian of China and its significance for cnidarian evolution. Nat. Commun. 2:442 doi: 10.1038/ncomms1457 (2011).